High-density magnetoresistive random access memory operating at ultralow voltage at room temperature The main bottlenecks limiting the practical applications of current magnetoresistive random access memory (MRAM) technology are its low storage density and high writing energy consumption. Although a number of proposals have been reported for voltage-controlled memory device in recent years, none of them simultaneously satisfy the important device attributes: high storage capacity, low power consumption and room temperature operation. Here we present, using phase-field simulations, a simple and new pathway towards high-performance MRAMs that display significant improvements over existing MRAM technologies or proposed concepts. The proposed nanoscale MRAM device simultaneously exhibits ultrahigh storage capacity of up to 88 Gb inch −2 , ultralow power dissipation as low as 0.16 fJ per bit and room temperature high-speed operation below 10 ns. Magnetoresistive random access memory (MRAM), because of its moderately fast access time and almost unlimited endurance, has offered a tantalizing application potential as next-generation non-volatile integrated memories [1] . However, mass production of MRAMs has long been hampered by their high writing energy from Ampère-current-induced magnetic field [2] , [3] . This would also cause severe cross-talk among neighbouring cells when miniaturizing the device size for higher storage capacity. One promising solution is to develop voltage-write MRAM devices [4] , that is, manipulating magnetization directly using electric voltage rather than current. Previous proposals include integrating a spin valve [5] or magnetic tunnel junction (MTJ) [6] unit onto a multiferroic layer (for example, Cr 2 O 3 (ref. 7 ) or BiFeO 3 (ref. 8 )), and more recently using ferroelectric (FE) oxide as the tunnel barrier as in a Fe/BaTiO 3 /(La,Sr)MnO 3 junction [9] where significant voltage control of tunnel magnetoresistance [6] was realized at rather low temperatures. Nonetheless, no existing proposals have so far achieved low voltage, high storage density and room temperature operation all at the same time. In this study, we illustrate a simple and new approach towards ultralow voltage-controlled MRAMs using phase-field simulations. We show that the proposed device is capable of achieving ultralow writing energy (less than 0.16 fJ per bit), room temperature (or even wider range) operation and high storage density (up to 88 Gb inch −2 ) all at the same time, associated with reliable thermal stability (quality factor over 40 at T =300 K) and comparable writing speed (sub-10 ns). 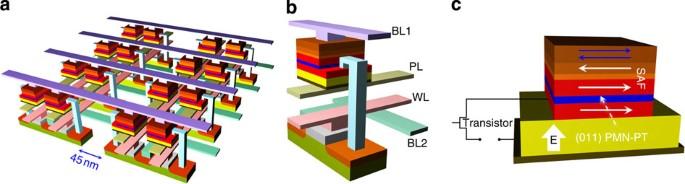Figure 1: High-density MRAM operating at ultralow voltage at room temperature. (a) Array design of the electric-field-controlled MRAM device on CMOS platforms. The space between neighbouring cells is taken as 45 nm, which is the typical channel length of its constituent MOS transistor. (b) Architecture of the 1-T(transistor)/1-magnetoresistive (MR) memory unit cell, where the writing voltage is applied between Bitline (BL)2 and Plateline (PL) controlled by Wordline (WL) connecting to the gate of the transistor. (c) Schematic of the basic building block, where a spin valve or magnetic tunnel junction is integrated onto a PMN-PT layer, upon the application of a perpendicular voltage bias controlled by the transistor. (From top to bottom): antiferromagnetic pinning layer, a synthetic antiferromagnetic tri-layer with a pinned layer and a reference layer separated by ultrathin non-magnetic spacer, tunnelling barrier/non-magnetic metallic layer, the magnetic-free layer, ferroelectric layer, and the bottom electrode. The arrows in the MR element denote the magnetization orientations. Ultralow voltage-controlled MRAM device structure Figure 1a illustrates one possible layout of a memory cell array, which builds on planar complementary metal-oxide-semiconductor (CMOS) platforms. As in normal MRAMs, it has a typical 1-T(transistor)/1-magnetoresistive(MR) element cell architecture ( Fig. 1b ), where the readout is accomplished by sensing the resistance change of the cell. However, the most remarkable feature is its ideal zero current, gate-controlled-write process (see Methods section for the operation time sequence), which is fast and extremely power-efficient. There are virtually no cross-talks among neighbouring cells. It has a simple structure, which is easier to manufacture than conventional MRAMs, due to the absence of extra current-carrying lines. The simplicity offers a great potential for realizing high storage capacity. The basic building block, incorporating a spin valve or MTJ unit onto a (011)-oriented perovskite FE (for example, lead magnesium niobate-lead titanate, PMN-PT) layer (or maybe (001)-oriented rhombohedral FE layer with spontaneous polarization along 〈111〉 directions), is shown in Figure 1c . An external electric voltage is perpendicularly applied to the PMN-PT layer triggered by the connecting transistor. This produces large anisotropic in-plane piezostrains [10] , which would be further imparted to its upper magnetic-free layer and induces a 90° in-plane magnetization rotation in the latter via the strain-mediated converse magnetoelectric coupling [11] , [12] . By operating the (011)-oriented PMN-PT layer below its FE coercive field, bistable in-plane piezostrains can be obtained, that is, the strain states can be maintained even when the applied voltages are switched off, as demonstrated by a permanent magnetization switching observed recently in polycrystalline Ni thin film grown on (011) PMN-PT [13] . This interesting bistable magnetization switching should bring greater design flexibility to the present voltage-controlled MRAM devices, that is, the non-volatility can be achieved not only by virtue of high-quality epitaxial magnetic thin films whereby the magnetocrystalline anisotropy serves as the potential barrier [3] , but also in polycrystalline and/or amorphous thin films, despite a little lower magnetoresistance ratio due to structural imperfections in the latter. Figure 1: High-density MRAM operating at ultralow voltage at room temperature. ( a ) Array design of the electric-field-controlled MRAM device on CMOS platforms. The space between neighbouring cells is taken as 45 nm, which is the typical channel length of its constituent MOS transistor. ( b ) Architecture of the 1-T(transistor)/1-magnetoresistive (MR) memory unit cell, where the writing voltage is applied between Bitline (BL)2 and Plateline (PL) controlled by Wordline (WL) connecting to the gate of the transistor. ( c ) Schematic of the basic building block, where a spin valve or magnetic tunnel junction is integrated onto a PMN-PT layer, upon the application of a perpendicular voltage bias controlled by the transistor. (From top to bottom): antiferromagnetic pinning layer, a synthetic antiferromagnetic tri-layer with a pinned layer and a reference layer separated by ultrathin non-magnetic spacer, tunnelling barrier/non-magnetic metallic layer, the magnetic-free layer, ferroelectric layer, and the bottom electrode. The arrows in the MR element denote the magnetization orientations. Full size image Compared with previous MRAM proposals [7] , [8] , [9] , the present voltage-write MRAM device is actuated at an ultralow voltage, as discussed below. Second, the strain-mediated magnetoelectric coupling offers a straightforward way to electrically manipulate the magnetization at room temperature, whereas the promising Fe/BaTiO 3 /(La,Sr)MnO 3 junction [9] is limited to low temperature. Moreover, our proposed voltage-write MRAM device has a much wider operation temperature range than the voltage-controlled MRAM that uses Cr 2 O 3 with its Néel temperature ( T N ~307 K) close to room temperature [7] . Third, the perpendicular writing voltage bias ( Fig. 1c ) makes it easy to integrate it with existing CMOS platforms ( Fig. 1a ) to fabricate nanoscale high-density memory devices. In contrast, multiferroic BiFeO 3 -based MRAMs demonstrated so far [8] require an in-plane actuation electric field. Such a transverse actuation voltage along the in-plane direction usually resorts to an interdigitized transducer patterning, which is typically of a micron size [14] , and intrinsically prohibits high storage capacity. This is also the case for the voltage-controlled MRAM using (001)-oriented FE layer [15] , [16] , [17] . Working and design principles of the device For illustration, we perform phase-field simulations of this electric-field-controlled MRAM device by choosing a (001) Ni film as the free layer. A spin valve comprising a synthetic antiferromagnetic layer ( Fig. 1c ) is considered as the upper MR element while an MTJ is also available. An initial uniform [010] magnetization is assumed for the Ni-free layer, which is exchange coupled to its upper reference layer. This direction can be set by annealing the device in a magnetic field. As described above, a perpendicular electric field E is applied to the bottom (011) PMN-PT layer to generate the anisotropic in-plane piezostrains [13] , subsequently inducing the in-plane magnetization rotation. By solving the Landau–Lifshitz—Gilbert (LLG) equation, both the macroscopic magnetization states and microscopic magnetic domain structure can be obtained (Methods section). We also performed a preliminary simulation to study the electric-field-induced magnetization switching in Ni/PMN-PT bilayer instead of the whole device. The simulation results agree well with corresponding experimental results [13] ( Supplementary Fig. S1 and Supplementary Note 1 ), demonstrating that this micromagnetic phase-field approach is valid. 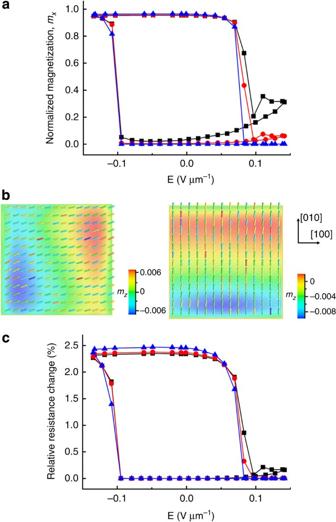Figure 2: Thickness-dependent switching behaviour. (a) Electric-field-induced magnetization rotation in the Ni-free layers with thicknesses of 35 nm (squares), 15 nm (circles) and 5 nm (triangles), respectively.mxindicates the the normalized magnetization in the in-plane [100] direction. The lateral size (length and width) is set as 64 nm. (b) Vector diagrams of the bistable magnetization distributions atE=0, that is,mx=0.9538 (left) and 0.0364 (right), in the 64×64×35 nm3Ni-free layer. (colour bar)mzindicates the normalized magnetization in the out-of-plane [001] direction. (c) Hysteric loops of relative device resistance change upon the perpendicular electric fields applied to the (011) PMN-PT layer, accompanied with the magnetization switching in the Ni-free layers with thicknesses of 35 nm (squares), 15 nm (circles) and 5 nm (triangles), respectively. By further introducing the dipole coupling between the Ni-free layer and its upper reference layer (equation (4) in Methods section), the thickness-dependent E -induced magnetization switching in the Ni-free layers are plotted in Figure 2a . As shown, bistable magnetization states are exhibited at E =0, for example, m x =0.9538 and 0.0364 for the 64×64×35 nm 3 Ni-free layer, corresponding to a magnetization rotation of about 70°. This is also directly illustrated by their magnetic vector diagrams shown in Figure 2b . Moreover, the magnetization– E curves become gradually flatter with the film thickness decreasing from 35 to 5 nm, along with a small increase in the maximum magnetization rotation around 5°. This can be attributed to the suppression of the out-of-plane magnetization component due to enhanced demagnetization in thinner magnetic thin films, which would in turn facilitate the in-plane magnetization rotation. The larger magnetization rotation further leads to a broader resistance change of the spin valve, as the device resistance is determined by the relative magnetization alignment, analytically expressed as [15] , Figure 2: Thickness-dependent switching behaviour. ( a ) Electric-field-induced magnetization rotation in the Ni-free layers with thicknesses of 35 nm (squares), 15 nm (circles) and 5 nm (triangles), respectively. m x indicates the the normalized magnetization in the in-plane [100] direction. The lateral size (length and width) is set as 64 nm. ( b ) Vector diagrams of the bistable magnetization distributions at E =0, that is, m x =0.9538 (left) and 0.0364 (right), in the 64×64×35 nm 3 Ni-free layer. (colour bar) m z indicates the normalized magnetization in the out-of-plane [001] direction. ( c ) Hysteric loops of relative device resistance change upon the perpendicular electric fields applied to the (011) PMN-PT layer, accompanied with the magnetization switching in the Ni-free layers with thicknesses of 35 nm (squares), 15 nm (circles) and 5 nm (triangles), respectively. Full size image Here R 0 denotes the device resistance with parallel magnetization configuration in the reference and free layer, and R MR the maximum magnetoresistance ratio, that is, the relative device resistance change between the parallel and antiparallel magnetization alignments. For illustration, R MR is taken as 7% for a normal spin valve [18] with giant magnetoresistance effect. Corresponding to the greater magnetization switching, increased maximum resistance changes are exhibited as indicated in Figure 2c . This may suggest the first design principle of such voltage-write MRAM device: the thinner, the better. However, growing ultrathin films requires more sophisticated processing control. Besides, the interface magnetic anisotropy contribution may lead to additional effect on the magnetization switching [19] , especially in ultrathin (several monolayers) films [20] , but is not considered herein regarding the robust magnetoelastic coupling of Ni as well as the large piezoelectric response of PMN-PT, which should in principle produce a large strain-mediated magnetoelectric response [19] . Nonetheless, based on the results in Figure 2 , 5 nm could be a well-compromised thickness for metallic Ni-free layer deposited on the PMN-PT. In particular, the actuation electric field required for the MRAM device is ultralow, that is, | E |<0.2 V μm −1 ( Fig. 2c ). As small lateral size of the spin valve is highly desirable for pursuing high storage density, we examine the lateral size effect of the free layer on the E -induced magnetization switching while fixing the film thickness at 5 nm. 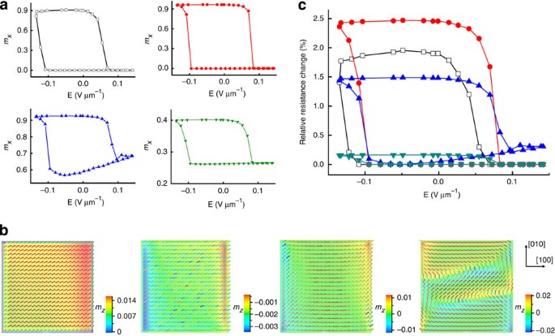Figure 3: Lateral size-dependent switching behaviour. (a) Electric-field-induced magnetization rotation in Ni layers with lateral sizes (length and width) of 32 nm (squares), 64 nm (circles), 128 nm (up triangles) and 192 nm (down triangles), respectively.mxindicates the normalized magnetization in the in-plane [100] direction. The free layer thickness is set as 5 nm. (b) Magnetic vector diagrams of the 5 nm Ni-free layers with lateral sizes of (from left to right) 32, 64, 128 and 192 nm, wheremx=0.9032, 0.9638, 0.9253 and 0.4014, respectively. (colour bar)mzdenotes the out-of-plane normalized magnetization component. As shown, the optimized lateral size cannot be too big or too small, otherwise the magnetization switching would be hampered either by formation of multi-domains or the enhanced lateral demagnetization. (c) Hysteric loops of relative device resistance change versus the applied electric field, accompanied with the magnetization switching in the Ni-free layers with lateral sizes of 32 nm (squares), 64 nm (circles), 128 nm (up triangles) and 192 nm (down triangles), respectively. As seen from Figure 3a , a square-shaped magnetization− E loop is exhibited even when the lateral size reduces to 32 nm, and hence it can be used for bistable memory implementation. This naturally leads to the second design principle of this E -controlled MRAM device: the smaller, the better. However, it cannot be considered as a generalized conclusion, as the complex magnetization distribution near the lateral edges would, to some extent, hamper the in-plane magnetization rotation when the lateral sizes are shrunken. This is evidenced by a moderate reduction of the maximal magnetization rotation when the lateral size decreases from 64 to 32 nm ( Fig. 3a ). One may refer to the magnetic vector diagrams in Figure 3b to compare the different magnetization distributions near the square edges. In addition, the deterioration of thermal stability with reduced free layer volume is another issue that will be discussed below. On the other hand, for the free layers with lateral size larger than 128 nm, the E -induced in-plane magnetization rotation would be significantly cancelled out by the presence of multi-domains (see the corresponding magnetic vector diagram in Fig. 3b ) driven by the demagnetization field in the lateral direction, and thus leads to much smaller relative resistance changes, as indicated in Figure 3c . It should be noted that the magnetization–resistance relationship in multi-domain-free layers might not exactly be described by equation (1), as different regions of magnetizations (namely, the magnetic domains) could separately contribute to the resistance change. Nevertheless, it is still rational to believe that the multi-domain-free layer generally shows a smaller maximum resistance change than its single-domain counterpart, except for those with very narrow lateral sizes. The latter will also hamper the magnetization switching and the resultant resistance change as discussed above. Thus, the Ni-free layer with a size of 64×64×5 nm 3 is likely a good choice for the experimental demonstration of such voltage-actuated MRAM device due to both large resistance change and thermal stability factor (see Figs 3c and 4 ). Figure 3: Lateral size-dependent switching behaviour. ( a ) Electric-field-induced magnetization rotation in Ni layers with lateral sizes (length and width) of 32 nm (squares), 64 nm (circles), 128 nm (up triangles) and 192 nm (down triangles), respectively. m x indicates the normalized magnetization in the in-plane [100] direction. The free layer thickness is set as 5 nm. ( b ) Magnetic vector diagrams of the 5 nm Ni-free layers with lateral sizes of (from left to right) 32, 64, 128 and 192 nm, where m x =0.9032, 0.9638, 0.9253 and 0.4014, respectively. (colour bar) m z denotes the out-of-plane normalized magnetization component. As shown, the optimized lateral size cannot be too big or too small, otherwise the magnetization switching would be hampered either by formation of multi-domains or the enhanced lateral demagnetization. ( c ) Hysteric loops of relative device resistance change versus the applied electric field, accompanied with the magnetization switching in the Ni-free layers with lateral sizes of 32 nm (squares), 64 nm (circles), 128 nm (up triangles) and 192 nm (down triangles), respectively. 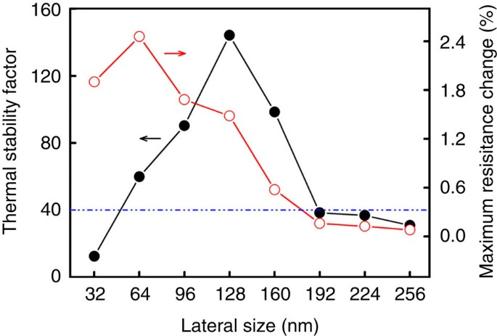Figure 4: Device thermal stability and maximum resistance change. The thermal stability factor (atT=300 K) and maximum resistance change of the present voltage-controlled MRAM device as a function of the lateral size (length and width) of its Ni-free layer. The free layer thickness is set as 5 nm. The dashed line shows the minimum thermal stability requirement for a reliable non-volatility of the MRAM device. Full size image Figure 4: Device thermal stability and maximum resistance change. The thermal stability factor (at T =300 K) and maximum resistance change of the present voltage-controlled MRAM device as a function of the lateral size (length and width) of its Ni-free layer. The free layer thickness is set as 5 nm. The dashed line shows the minimum thermal stability requirement for a reliable non-volatility of the MRAM device. Full size image The device thermal stability and power consumption The thermal stability factor is defined as F / k B T , where F = f barrier V f is the energy barrier that separates the two stable magnetization states ( V f denotes the volume of the free layer, k B the Boltzmann constant and T the temperature set as 300 K). To ensure a reliable non-volatility, a thermal stability factor of higher than 40 is normally required [3] . While common MRAMs rely on the intrinsic magnetic anisotropy energy (for example, the magnetocrystalline anisotropy) to retain the magnetization state, the energy barrier mostly results from the extrinsic elastic strain stimuli in the present proposal, which eliminates the specific crystal structure [3] , [15] requirements for the free layer and offers more design flexibility. The potential barrier energy f barrier can be estimated by calculating the free energy difference between the two stable magnetization states at E =0. Similarly, fixing the film thickness to 5 nm, the lateral size dependence of the thermal stability factor is given in Figure 4 , with their corresponding relative resistance changes shown for comparison. From the plots, it can be clearly seen that the free layer with lateral sizes from 64 to 160 nm exhibit both sufficient thermal stability and comparable resistance change, although the latter two attributes appear not possible to be simultaneously optimized. Nevertheless, the results indicate that Ni films with lateral sizes of between 64 and 160 nm, and thickness of about 5 nm, should be suitable for application as the free layers of such novel MRAM devices. If further reducing the lateral size for higher storage density, then efforts should be made to compensate the concomitant loss of the thermal stability, as well as the reduction of the maximum resistance change due to the hampered in-plane magnetization rotation. As mentioned at the beginning, the ultralow power consumption, resulting from both the inherent energy efficiency of electrical switching [21] and its ultralow actuation voltage, is the most advantageous quality of the present ultralow electric-voltage-controlled MRAM, far superior to any other existing or emerging MRAM technologies. Figure 2c shows such a small E writing window from about −0.13 to 0.1 V μm −1 . That means, if using a 2-μm PMN-PT thick layer, an ultralow voltage of about 0.26 V would be sufficient for the device operation. This operation voltage is much lower than those reported previously in the proof-of-concept experiments [14] , [22] . For further illustration, we estimate the writing energy as [1] ½ P r SV in terms of charging the FE capacitor, where P r , S and V denote the remnant polarization, electrode area and the operation voltage, respectively. In this case, an extremely low writing energy of around 0.16 fJ per bit can in principle be obtained by taking P r =30 μC cm −2 (ref. 13 ), S =0.0041 μm 2 (for a 64×64 nm 2 free layer electrode) and V =0.26 V. This energy consumption is drastically lower than 70 pJ per bit for conventional MRAMs [1] , and even orders of magnitude lower than 0.1 pJ in the state-of-the-art spin-transfer-torque (STT) MRAM technology [23] , which is deemed as the most reachable solution for next-generation MRAMs, and is currently under intense industrial interests. As this low actuation electric field remains below the FE coercive field of the PMN-PT (approximately ±0.2 V μm −1 (ref. 13 )), the fatigue problem that FEs (including multiferroic BiFeO 3 ) typically suffer from repetitive polarization reversal can also be greatly relieved. This should allow an effective alleviation of the energy loss and improvement of device reliability. Furthermore, the dielectric breakdown vulnerability of the present device can be avoided as the write operating voltage, far below the dielectric breakdown threshold of the PMN-PT (>10 V μm −1 (ref. 24 )), is applied only on the PMN-PT layer. This structural feature of the present device is different from that in STT-RAMs, where the write and read current flow across the whole device and share the same tunnel. Writing speed and storage capacity Another important performance attribute of the voltage-controlled MRAM device is the writing speed, which typically takes less than 10 nanoseconds (ns) or with a possibility of sub-1 ns (see the write-time estimation and corresponding electric-field-induced dynamic magnetization switching in the Methods section). This operation speed is significantly higher than conventional magnetic-write MRAM (around 20 ns (ref. 1 )), while comparable with the STT-MRAM devices (~3 to 10 ns (ref. 25 )). Finally, the fully gate voltage-controlled operation allows a good compatibility of the present device with current CMOS platforms, opening up possibilities for ultrahigh densities. For instance, assuming a typical channel length of 45 nm for the bottom transistor ( Fig. 1a ) and the lateral size of 64 nm for the upper ME spin valve (or MTJ)/PMN-PT heterostructure, a storage density of around 88 Gb inch −2 can in principle be realized, challenging traditional NAND Flash memory on mass data storage applications [26] . For comparison, the properties obtained in the present device prototype are summarized in Table 1 , including several other existing room temperature non-volatile memory technologies. Table 1 Comparison of room temperature non-volatile memory technologies. Full size table We have demonstrated a simple and new approach towards ultralow voltage-controlled MRAMs. The present voltage-controlled MRAM device can be fabricated on CMOS platforms, wherein the basic building block comprises of a spin valve or MTJ MR element grown on a (011) PMN-PT layer. Without necessarily requiring epitaxial growth of the magnetically free layer, simply utilizing a specifically engineered FE layer with voltage-induced bistable anisotropic in-plane piezostrains, one can realize most important attributes required by modern MRAM technology at the same time. Therefore, we expect our finding will stimulate future experimental and engineering efforts on developing such an electric-voltage-controlled device, which has superiorities over the previous device paradigms [7] , [8] , [9] , [14] , [22] . The present device proposal represents a simple pathway to realizing high-density, low voltage-controlled MRAM applications at room temperature, either as standalone/embedded memories or logic circuits. 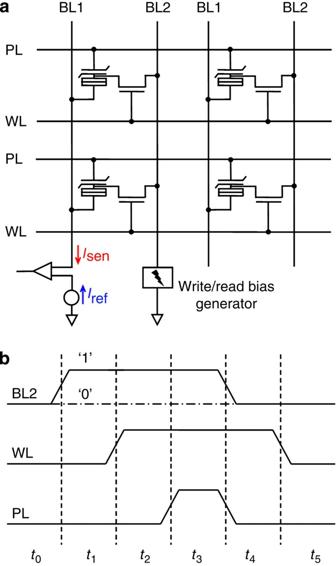Figure 5: Device operation illustration. (a) Cell array image of the voltage-controlled MRAM device. BL, PL and WL stands for bitline, plateline and wordline, respectively. (b) Illustration of writing time sequence. The state '1' is written at the time stage 't2', where the voltages in BL2 and PL are in high and low level, respectively. Writing a '0' (corresponding to the dash dot line in the row BL2) is accomplished at the time stage 't3' in a similar manner, but the BL2 and PL are in reverse polarities. Operation time sequence of the device As seen in Figure 5a , the write voltage bias is applied between the Bitline (BL2) and the plateline (PL), which is controlled by the Wordline (WL) connecting to the gate of transistor. Corresponding writing time sequence is shown in Figure 5b . While to read, the sensing current ( I sen ) travels through the transistor and the MR element from BL2 to BL1, to generate the high and low output voltages, that is, Figure 5: Device operation illustration. ( a ) Cell array image of the voltage-controlled MRAM device. BL, PL and WL stands for bitline, plateline and wordline, respectively. ( b ) Illustration of writing time sequence. The state '1' is written at the time stage ' t 2 ', where the voltages in BL2 and PL are in high and low level, respectively. Writing a '0' (corresponding to the dash dot line in the row BL2) is accomplished at the time stage ' t 3 ' in a similar manner, but the BL2 and PL are in reverse polarities. Full size image where R MOS is the resistance of the transistor; R high and R low denote the bistable resistance states of the MR element resulting from the voltage-induced magnetization switching in the magnetic-free layer. The reference current ( I ref ) is set to a specific value so that the corresponding reference voltage ( V R ) is ideally between V high and V low . Introduction to the phase-field method In the phase-field approach, the magnetic domain structure is described by the spatial distribution of the local magnetization vectors M = M s m = M s ( m x , m y , m z ), where M s and m i ( i = x , y , z ) represent the saturation magnetization and the direction cosine, respectively. The temporal evolution of the magnetization configuration and thus the domain structure is governed by the LLG equation, that is, where γ 0 and α are the gyromagnetic ratio and the damping constant, respectively, and H eff the effective magnetic field, given as Here μ 0 denotes the vacuum permeability, and F tot is the total free energy of the magnetic-free layer, where F mc , F ms , F ex and F elas are the magnetocrystalline anisotropy, magnetostatic, magnetic exchange and elastic energy, respectively. F dip describes the ferromagnetic-type dipole coupling between the free layer and its upper reference layer, given as for an initial [010] magnetization; H dip is the effective interlayer dipole coupling field taken as 40 Oe for illustration (see more discussions on the influence of H dip in Supplementary Fig. S2 and Supplementary Note 2 ). The magnetostatic energy F ms can be written as, where H d denotes the stray field arising from the long-range magnetization interactions in the system, given as being the average magnetization field). To incorporate the influence of the specific sample geometric size, a finite-size magnetostatic boundary condition is used for obtaining F ms , with the demagnetization factors N in the magnetostatic energy calculated numerically [27] . The mathematical expressions of F mc and F ex for cubic ferromagnets are the same as those given in refs 11 and 27 . The elastic energy F elas can be written as, where e ij is elastic strain, c ijkl the elastic stiffness tensor and ɛ ij the total strain that can be represented as the sum of homogenous and heterogeneous strains following Khachaturyan's mesoscopic elastic theory [28] , The heterogeneous strain η ij is defined in such a way so that , and the homogeneous strain describes the macroscopic shape change of the magnetic thin film. Specifically, and , namely, the homogeneous strains along the two in-plane crystal axes, can be expressed as, Here and denote the contribution from the piezoelectric transformation of the bottom PMN-PT layer, which we directly use the experimental data reported in ref. 13 as the input. We also assume that the PMN-PT layer is much thicker than the upper magnetic film to ensure a full strain transfer [29] . ɛ 0 is the biaxial residual strain resulting from the lattice and/or thermal mismatch. For a polycrystalline magnetic film deposited at room temperature, ɛ 0 almost equals zero; while for an epitaxial film, it depends on the specific substrate as well as the growth condition [30] . Note that ɛ 0 should exert no influence on the in-plane magnetization rotation ( Supplementary Fig. S3 and Supplementary Note 3 ), although it does have effects on the specific magnetic domain structure in the free layer [31] . Here it is taken as −0.5% for illustration. represents the stress-free strain describing the stress-free deformation of a cubic ferromagnet associated with the local magnetization change, where λ 100 and λ 111 are the magnetostrictive constants. By further considering a mixed boundary condition for the film-substrate system [32] , F elas can be calculated by combining Khachaturyan's theory [28] with the Stroh's formalism of anisotropic elasticity [33] . The temporal evolution of the local magnetization and thus the domain structures are obtained by numerically solving the LLG equation using the semi-implicit Fourier spectral method [34] . To illustrate the Ni-free layer with a size of 64×64×35 nm 3 , the magnetic film is discretized into a three-dimensional array of cubic cells of 64Δ x ×64Δ y ×35Δ z , with the grid size Δ x =Δ y =Δ z =1 nm in real space accordingly. A three-dimensional finite-size boundary condition is considered to calculate the geometric-size-related magnetostatic anisotropy energy as mentioned above. By varying the simulation zone size and/or the grid size, magnetic-free layers with different geometric sizes (for example, thickness and lateral size, see Figs 2 and 3 ) can then be treated. Each simulation starts with an initial [010] magnetization distribution accordingly and proceeds for long enough time to ensure a stabilized magnetization distribution, with a normalized time step Δ τ =0.01. The Landau, elastic and magnetic parameters used for simulation are described in the literature [11] , [35] . Write-time estimation Such electric-field-controlled MRAM device can at least allow a sub-10 ns writing, which is much faster than conventional magnetic-field-switched MRAM (about 20 ns (ref. 1 )) and comparable with practical STT-MRAM devices (about 3–10 ns (ref. 25 ). First, based on LLG equation, the average magnetization switching time is estimated as about 0.95 ns for magnetic-free layers with various lateral sizes (the thickness is set as 5 nm likewise), typically allows a GHz operation frequency. The details about such electric-field-induced dynamic switching will be shown below. The dynamic parameters used in LLG equation are: Damping constant: α =0.038 (experimental measurement for 5 nm Ni films [36] ). Gyromagnetic ratio: γ 0 =− 2.42×10 5 m (A s) −1 (using g= 2.21 from ref. 36 ). However, there are other factors that can affect practical writing speed such as the time the PMN-PT layer produces the piezostrain (that is, the electric polarization switching time with the associated strain), and the time for the strain transfer across the Ni/PMN-PT interface (we tentatively do not consider the influence of buffer layer that might be required for epitaxial growth) and getting its mechanical equilibrium. For the first part, note that polarization normally switches much faster than the magnetization (the switching time is usually below 10 ns (ref. 37 ). That is also the reason why a FeRAM takes less time to write information compared with common MRAMs (see Table 1 ). Moreover, it is worth noting that there is no full polarization reversal in the PMN-PT layer in our case, as the actuation electric field (−0.13 to 0.1 V μm −1 ) remains below the FE coercive field (approximately ±0.2 V μm −1 (ref. 13 )), which further reduces the switching time. Also for a given polarization distribution, one can assume that the FE layer undergoes piezoelectric deformation and reaches its mechanical equilibrium almost instantaneously, as the mechanical relaxation of an elastic field is even faster than that of a polarization [38] . Moreover, it should also be noted that although higher actuation electric field bias could lead to faster electric polarization switching in the FE layer to some extent, the overall device switching speed would not be significantly enhanced due to the inherent piezostrain-induced magnetization switching. Specifically, the maximal remnant piezostrain at zero electric field ( E =0) almost remains stable when the write E -field is increased from 0.13 to 0.2 V μm −1 (ref. 13 ). This feature is quite different from normal STT-RAM devices where faster switching could be facilitated by imposing higher operating voltage, while unavoidably exhibits higher vulnerability to dielectric break down as well. As for the pizeostrain transfer time τ , we give a rough estimation on this short time span [39] , where d 1 and d 2 are the thicknesses; and v 1 and v 2 the velocity of sound in the FM and FE layer, respectively. For illustration, assuming d 1 =5 nm (the Ni film thickness), d 2 =2 μ m for the PMN-PT layer and v 1 ≈ v 2 =3,000 m s −1 (it is well known that the speed of sound varies from substance to substance, but generally it travels very fast in solids, say, about 5,120 m s −1 in iron at 293 K), then we have τ ≈0.67 ns. Note that we have considered the stress wave that covered the whole device system, but the effective mechanical coupling is more likely to be confined in a closer vicinity of the interface, which means the strain transfer time could be even shorter. Overall, although the practical strain mediation situation could be far more complex than the simple model described above (such as the influences of the mechanical resonance frequency, and the Resistor-Capacitor time constant associated with charging the FE capacitor, see related discussion in ref. 40 ), it is rational to consider the stress to be applied almost instantaneously to the FM film [40] . Thus in total, the theoretical writing time of such electric-field-controlled MRAM device can be estimated to be about 1.62 (=0.95+0.67) ns, well within a 10 ns range required by future applicable MRAM technologies [41] . This result is comparable with the results reported for other related device proposals with similar strain-mediated electric-write procedure, such as multiferroic logic [40] , [42] or nanowire memory [43] devices, which use either Terfenol-D [40] (Ni (ref. 42 )) particles, or FeGa (ref. 43 ) nanowires attached to a commercial Pb(Zr,Ti)O 3 layer, all with an estimated operation time less than 10 ns. Electric-field-induced dynamic magnetization switching The combination of phase-field model with micromagnetic simulation here in this paper allows us to go beyond the previous macro-spin model used for single-domain magnets [40] , [42] . Indeed, the free layer does not always behave as a single macro-spin when the lateral sizes exceed a certain critical value (possibly around 128 nm, see Fig. 3b ). 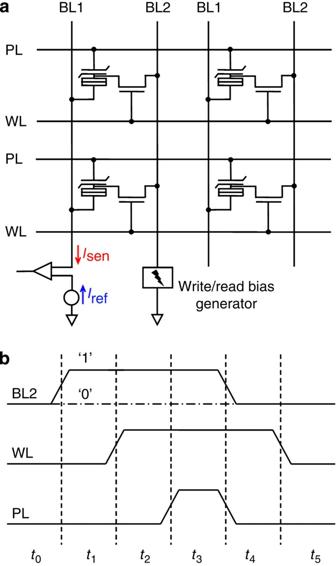Figure 6: Electric-field-induced dynamic magnetization switching. (a) Time-dependent electric-field-induced magnetization switching in 64×64×5 (squares) and 224×224×5 nm3(circles) Ni-free layers, corresponding to the higher remnantmxatE=0 (seeFig. 3a). For simplicity, the piezoelectric stress is considered to be applied to the Ni film instantaneously. (b) Snapshots of the magnetization vector diagrams in 64×64×5 nm3(top) and 224×224×5 nm3(bottom) Ni-free layers at (from left to right)t=0.13, 0.64, 0.90 and 1.02 ns, respectively. The arrows and the dashed curves are the eye guides for the coherent magnetization rotation and domain-wall motion processes in single-domain 64×64×5 and multi-domain 224×224×5 Ni films, respectively. For illustration, Figure 6a shows the time-dependent electric-field-induced magnetization switching processes in 64×64×5 and 224×224×5 nm 3 Ni-free layers, where the films are in single-domain and multi-domain states, respectively. As seen, the dynamic magnetization switching process exhibit a typical processional rotation feature (see the fluctuations of m x in Fig. 6a after t =0.77 ns, governed by LLG equation) in single-domain 64×64×5 nm 3 Ni films. By contrast, the 224×224×5 nm 3 Ni films present a much flatter magnetization switching by virtue of domain-wall motion (see the illustrations in Fig. 6b ), which is common in multi-domain magnetic thin films [44] . Note that the normalized magnetization m x does not eventually turn to unity due to the cancelling out of the magnetic vectors along the [100] direction. Figure 6: Electric-field-induced dynamic magnetization switching. ( a ) Time-dependent electric-field-induced magnetization switching in 64×64×5 (squares) and 224×224×5 nm 3 (circles) Ni-free layers, corresponding to the higher remnant m x at E =0 (see Fig. 3a ). For simplicity, the piezoelectric stress is considered to be applied to the Ni film instantaneously. ( b ) Snapshots of the magnetization vector diagrams in 64×64×5 nm 3 (top) and 224×224×5 nm 3 (bottom) Ni-free layers at (from left to right) t =0.13, 0.64, 0.90 and 1.02 ns, respectively. The arrows and the dashed curves are the eye guides for the coherent magnetization rotation and domain-wall motion processes in single-domain 64×64×5 and multi-domain 224×224×5 Ni films, respectively. Full size image How to cite this article: Hu, J.-M. et al . High-density magnetoresistive random access memory operating at ultralow voltage at room temperature. Nat. Commun. 2:553 doi: 10.1038/ncomms1564 (2011).